Direct biological fixation provides a freshwater sink for N2O Nitrous oxide (N 2 O) is a potent climate gas, with its strong warming potential and ozone-depleting properties both focusing research on N 2 O sources. Although a sink for N 2 O through biological fixation has been observed in the Pacific, the regulation of N 2 O-fixation compared to canonical N 2 -fixation is unknown. Here we show that both N 2 O and N 2 can be fixed by freshwater communities but with distinct seasonalities and temperature dependencies. N 2 O fixation appears less sensitive to temperature than N 2 fixation, driving a strong sink for N 2 O in colder months. Moreover, by quantifying both N 2 O and N 2 fixation we show that, rather than N 2 O being first reduced to N 2 through denitrification, N 2 O fixation is direct and could explain the widely reported N 2 O sinks in natural waters. Analysis of the nitrogenase ( nifH ) community suggests that while only a subset is potentially capable of fixing N 2 O they maintain a strong, freshwater sink for N 2 O that could be eroded by warming. Nitrous oxide (N 2 O) is a potent climate gas, with ~273 times the global warming potential of carbon dioxide (CO 2 ) [1] and strong ozone-depleting properties [2] . The atmospheric concentration of N 2 O continues to rise through the use of nitrogen-based fertilisers, fossil fuel combustion, biomass burning and sewage discharge [3] and has already increased by approximately 20% since 1750 [4] . Not surprisingly, given its atmospheric potency, research to date has focused on these N 2 O sources with N 2 O sinks being relatively understudied [5] , [6] , [7] . The few studies reporting on both N 2 O sources and sinks [8] , [9] , [10] , [11] often simply document the sinks as concentrations below that expected for water (marine or freshwater) at equilibrium with the atmosphere and the true mechanism behind this N 2 O deficit remains largely unknown. In terrestrial and aquatic environments, N 2 O can be produced from both microbial nitrification [12] either via hydroxylamine oxidation (NH 4 + → NH 2 OH → N 2 O), or hybrid formation (NO 2 − + NH 2 OH → N 2 O) [13] , and incomplete denitrification (NO 3 − → NO 2 − → NO→ N 2 O[ \(\to\) N 2 ]) [14] . Where oxygen is limiting and/or completely absent, N 2 O can be further reduced to N 2 in the last step of microbial denitrification (N 2 O→N 2 ) that is typically mediated by facultative anaerobic bacteria [14] , [15] . As such, any undersaturation – indicating a sink for N 2 O – as observed in some waters has routinely been attributed to that last step in denitrification. However, such N 2 O undersaturation has typically been reported in well-oxygenated, shallow freshwaters [8] , [9] , [10] , [16] , [17] , [18] , [19] , [20] , [21] (down to 13% of air equilibration, typically ~70–100%) and surface-ocean-waters [5] , [11] , [22] , [23] , [24] , [25] , [26] , [27] , [28] (down to 34%, typically ~90%) where canonical denitrification is unlikely to explain any undersaturation in N 2 O. While N 2 O consumption by denitrification has been reported in both anoxic and oxic-to-anoxic transitioning waters in the Eastern Tropical North Pacific [6] , the reasons for N 2 O undersaturation in general remain poorly understood, with many instances of N 2 O undersaturation remaining unaccounted for [8] , [9] , [10] , [19] , [20] , [21] or simply being dismissed as analytical artifacts [24] , [29] . Further, as N 2 O sources generally increase at higher concentrations of ammonium and nitrate (i.e., fixed, bio-available N) [8] , [25] , any potential undersaturation in N 2 O could be masked by stronger production of N 2 O from nitrification and denitrification. This might explain why many accounts of N 2 O undersaturation have been reported in N limited environments [5] , [9] , [19] , [21] , [22] . In recent years, evidence has been presented for an additional pathway to denitrification for N 2 O reduction, namely – N 2 O dependent N fixation – that has been reported for pure cultures of marine Trichodesmium and Crocosphaera [5] . N 2 O fixation has also been reported in the surface waters of the Eastern Tropical South Pacific [5] , [23] , where the measured N 2 O fixation activity could contribute some (0.2 – 60%) of the total N 2 O reduction [5] . As long ago as 1954, it was shown [30] that 15 N 2 O could be assimilated by soybean root nodules with activity comparable to 15 N 2 assimilation. These findings show that N 2 O fixation (e.g. N 2 O→NH 4 + ) represents an alternative N 2 O reduction pathway to the terminal step in denitrification (N 2 O→N 2 ) that may explain some of the undersaturation reported for N 2 O. Within the widespread accounts of N 2 O undersaturation found in well-oxygenated waters, only a few studies mentioned the possibility of N 2 O fixation [5] , [22] , [23] and it is not widely acknowledged. Primary production and N 2 fixation are tightly coupled in N-limited ecosystems [31] . Some early studies (1952–1986) showed that N 2 O is a competitive inhibitor for N 2 fixation and it could also be a substrate for the enzymatic nitrogenase complex [32] , [33] , [34] , [35] , indicating that N 2 O fixation (e.g. N 2 O→NH 4 + ) may be related to N 2 fixation (N 2 →NH 4 + ). Further, with its N≡N bond N 2 fixation has a high activation energy (~1 to 2 eV vs. 0.65 eV and 0.32 eV for respiration and photosynthesis, respectively) [36] , [37] which makes fixing N 2 in the cold energetically unfavourable. As a consequence, the abundance of diazotrophs has been shown to decrease as temperatures decline [36] . In contrast, the energy required to fix N 2 O (Eq. 1 , Δ G defined for freshwater at 10 °C, see Supplementary Text 1 ) is lower than that for N 2 (Eq. 2 ) and being able to fix N 2 O could confer an ecological advantage to some microbes either in the cold or when resources (light or reduced substrates) in general are limiting. [ 0.5N_2O+1.5H_2O→1NH_3+1O_2                Δ G=+ 247kJ                 (per NH_3) ]
 (1) 
    [ 0.5N_2+1.5H_2O→ 1NH_3+0.75O_2                   Δ G=+ 291kJ                    (per NH_3) ]
 (2) While the ~18% energy saving for fixing N 2 O versus N 2 is seemingly modest, it is comparable to the recognised 21% saving delivered by assimilating NO 3 − (Eq. 3 ) rather than fixing N 2 (ref. [38] ) (see Supplementary Text 1 ). [ NO_3^-+3H^++2e^-→ 1NH_3+1.5O_2                    Δ G=+ 241kJ                     (per NH_3) ]
 (3) With both the last step in denitrification (N 2 O→N 2 ) and N 2 O fixation (N 2 O→NH 4 + ) providing sinks for N 2 O it is ecologically important to distinguish between these two parts of total N 2 O reduction. Further, any genuine direct N 2 O fixation (N 2 O→NH 4 + ) needs to be distinguished from indirect N 2 O fixation i.e., that which could occur after the initial reduction of N 2 O to N 2 (N 2 O→N 2 →NH 4 + ). Despite the few studies [5] , [23] , [30] documenting N 2 O fixation so far, to the best of our knowledge, there has been no characterisation of N 2 O fixation in relation to canonical N 2 fixation through the dual use of 15 N 2 O and 15 N 2 in natural communities. In 2005, we set up 20 experimental ponds (each with 1 m 3 water volume, 0.5 m depth) in East Stoke, Dorset, UK, to experimentally study the whole-ecosystem effects of climate warming [39] , [40] , [41] . Here, however, we exploited the fact that our experimental ponds are also N-limited [41] , being fed only by rain water, to characterise any potential N 2 O fixation in a controlled, experimental system. Despite being artificial, the ponds have well-established freshwater ecosystems [39] , [40] , [41] , [42] with diverse cyanobacteria communities [42] , among which some Nostocales [43] and Oscillatoriales [44] are known to fix N 2 . Here, we show that the ponds are undersaturated in both N 2 and N 2 O and further hypothesise that the pond communities fix both gases to support primary production. Then, due to the different energy demands of N 2 and N 2 O fixation, we hypothesise that the two processes will respond differently to temperature. We use incubations with pond biomass and 15 N 2 and 15 N 2 O stable isotope techniques to quantify their fixation activity, distinguish direct from indirect N 2 O fixation and characterise the temperature dependence of each N-fixing process. Finally, with no known freshwater candidates for N 2 O fixation to date, we explore the recognised N 2 fixing community in relation to N 2 O fixation. We ask whether: 1, is N 2 O fixation mediated by the total nitrogenase ( nifH ) community simply in relation to the relative availability of N 2 O to N 2 ; or 2, is N 2 O fixation preferentially mediated by a subset of the nifH community? Contrasting seasonalities in undersaturation for N 2 and N 2 O Concentrations of dissolved N 2 O and N 2 were both significantly below atmospheric equilibration ( p < 0.001, Fig. 1a ) and the ponds are sinks for both atmospheric N 2 O and N 2 . Overall, N 2 O was more under-saturated than N 2 ( p < 0.001, t = −17.5, d.f. = 240.6, two-sided, Fig. 1a ), with a mean value of 79.1% ± 1.1% (mean ± s.e., as below) of air saturation compared to 98.5% ± 0.2% for N 2 . 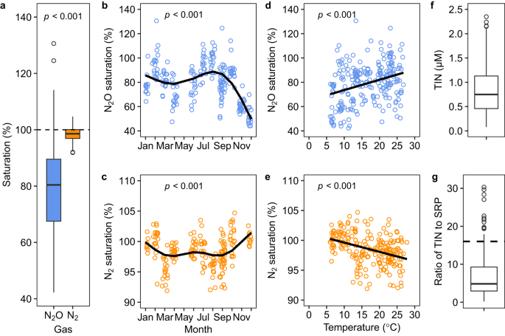Fig. 1: Seasonal and overall levels of N2O and N2saturation in the ponds. aBox-whisker plots showing overall that the saturation of N2O was lower than that for N2in the ponds (p< 0.001, two-sided, Supplementary Table1). The dashed line denotes 100% atmospheric equilibrium for the gases.b,cshow the saturation in N2O had a different seasonal pattern compared to N2(Note the different scales on the y-axes). The solid lines inbandcrepresent the best fitting GAMM models (two-sided, Supplementary Table1).dN2O saturation increased at higher temperatures while, in contrast,eN2saturation declined. The lines indandeare simple first-order linear regressions (two-sided).fOverall concentration of total inorganic nitrogen (TIN) in the ponds (n= 213 samples for 11 months in 20 ponds).gThe ratio of TIN to soluble reactive phosphorous (SRP) in the ponds (n= 168 samples for 11 months for 20 ponds, SRP data omitted below the detection limit). The dashed line ingdenotes the Redfield ratio of N to P of 16:1. Each box ina,fandgshows the 25th to 75th percentiles, horizontal lines the median, open circles denote outliers and whiskers extend to 1.5 times the interquartile range.n= 230 andn= 215 samples for N2O and N2saturation, respectively, for 20 ponds, in 11 months from November 2019 to April 2022 (see Supplementary Table2). Furthermore, the seasonality in N 2 O saturation was far more pronounced than for N 2 (Best fitting Generalised Additive Mixed Models, GAMMs, Supplementary Table 1 ), with a strong minimum for N 2 O in December and maximum saturation in summer (Fig. 1b ). Conversely, N 2 saturation peaked in winter and was lower in spring and summer (Fig. 1c ). Fig. 1: Seasonal and overall levels of N 2 O and N 2 saturation in the ponds. a Box-whisker plots showing overall that the saturation of N 2 O was lower than that for N 2 in the ponds ( p < 0.001, two-sided, Supplementary Table 1 ). The dashed line denotes 100% atmospheric equilibrium for the gases. b , c show the saturation in N 2 O had a different seasonal pattern compared to N 2 (Note the different scales on the y-axes). The solid lines in b and c represent the best fitting GAMM models (two-sided, Supplementary Table 1 ). d N 2 O saturation increased at higher temperatures while, in contrast, e N 2 saturation declined. The lines in d and e are simple first-order linear regressions (two-sided). f Overall concentration of total inorganic nitrogen (TIN) in the ponds ( n = 213 samples for 11 months in 20 ponds). g The ratio of TIN to soluble reactive phosphorous (SRP) in the ponds ( n = 168 samples for 11 months for 20 ponds, SRP data omitted below the detection limit). The dashed line in g denotes the Redfield ratio of N to P of 16:1. Each box in a , f and g shows the 25th to 75th percentiles, horizontal lines the median, open circles denote outliers and whiskers extend to 1.5 times the interquartile range. 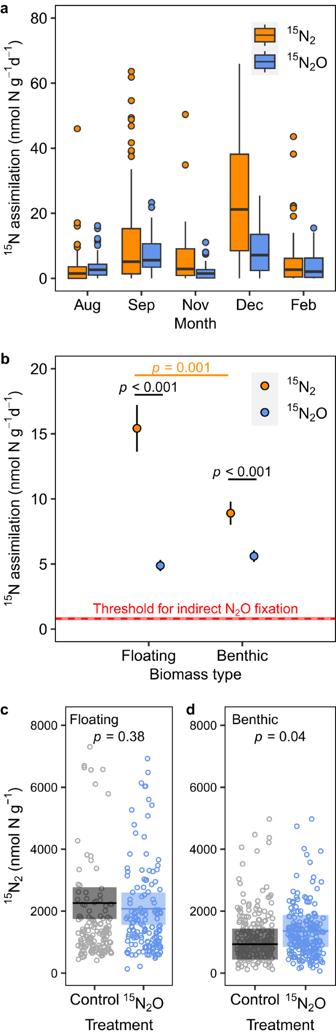Fig. 2: Evidence for the direct assimilation of15N into biomass from either15N2or15N2O. 15N assimilated into biomass from either15N2or15N2O in different months.aEach box shows the 25th to 75th percentiles, horizontal lines the median, open circles denote outliers, and whiskers extend to 1.5 times the interquartile range.bRates of15N2assimilation were higher than for15N2O assimilation in both biomass types. The red dashed line marks the upper threshold for indirect15N assimilation if15N2O was first reduced to15N2prior to assimilation (see Table1), red shaded area 95% C.I. Data plotted are means ± s.e. Yellow: difference between floating and benthic biomass with15N2(p= 0.001, two-sided),black: difference between15N2and15N2O in floating or benthic biomass (p< 0.001, two-sided). To exclude extreme outliers the data plotted inaandbare 95% of the dataset (2.5–97.5% percentiles). Data inaandbwere collected in 5 calendar months for 2 biomass types from 8 to 10 ponds per sampling date (n= 303 andn= 322 incubations for15N2and15N2O treatments, respectively).cNo significant production of15N2from15N2O in the floating biomass, butdsignificant production of15N2in the benthic biomass (p= 0.04, two-sided). The horizontal line is the mean and shaded area 95% C.I. (n= 351 incubations for both controls and15N2O treatments). n = 230 and n = 215 samples for N 2 O and N 2 saturation, respectively, for 20 ponds, in 11 months from November 2019 to April 2022 (see Supplementary Table 2 ). Full size image The concentrations of dissolved inorganic nutrients (nitrite, NO 2 − ; nitrate, NO 3 − ; ammonium, NH 4 + , and soluble reactive phosphorus, SRP) were low in the ponds, with NO 2 − , NO 3 − and NH 4 + often at or below the limit of detection. The concentration of total inorganic nitrogen (TIN as the sum of NO 2 − , NO 3 − and NH 4 + ) was 0.85 ± 0.03 µM across all sampling months (Fig. 1f ). SRP concentrations were 0.14 ± 0.01 µM, on average, and, at 5 to 1, the median N to P ratio was markedly lower than Redfield [45] (16 to 1), indicating primary production in the ponds to be N limited (Fig. 1g ). As the ponds were N-limited, primary production must be sustained largely by N fixation (and any unknown atmospheric N deposition), which may have resulted in the undersaturation of N 2 and N 2 O in the ponds. Interestingly, N 2 O saturation increased with water temperature ( p < 0.001, Fig. 1d ), suggesting relatively higher net reduction of N 2 O in the cold ( see Supplementary Fig. 1 for concentration data). Whereas N 2 saturation showed the opposite pattern, with relatively more net N 2 reduction at higher temperatures ( p < 0.001, Fig. 1e ) in spring and summer. Moreover, the saturation of dissolved O 2 in the ponds (at the same depth where the samples for N 2 and N 2 O were collected) was generally around air-equilibration (104.8% ± 1.8%, median 99.6%), with N 2 saturation decreasing at higher O 2 saturations, while N 2 O saturation increased with higher O 2 saturation (Supplementary Fig. 2 ). Oxygen saturation was positively correlated with temperature (Supplementary Fig. 2c ), probably due to higher temperatures in spring and summer promoting primary production. Therefore, maximum N 2 undersaturation was probably related to higher primary production in spring and summer [40] . The negative and positive correlations between N 2 or N 2 O and O 2 respectively, indicated different controls for the reduction of N 2 and N 2 O. N 2 O and N 2 fixation by biomass in the ponds To rationalise the undersaturation in both N 2 O and N 2 in our ponds, we measured fixation of either 15 N 2 O or 15 N 2 (at a range of temperatures, see below) by biomass collected from the ponds (Supplementary Fig. 3 ). We found 15 N assimilated into biomass from either 15 N 2 or 15 N 2 O in the majority of our incubations (87%, 572 out of 658 incubations, Fig. 2a ), with higher rates of 15 N assimilation with 15 N 2 than for 15 N 2 O with both floating and benthic biomass ( p < 0.001, t = 6.5, d.f. = 369.7, two-sided, Fig. 2b ). On average, 11.5 ± 0.9 and 5.3 ± 0.3 nmol g −1 d −1 (mean ± s.e.) of 15 N were assimilated into biomass with either 15 N 2 or 15 N 2 O, respectively (Fig. 2b ). The rate of 15 N 2 assimilation was higher in the floating than the benthic biomass ( p = 0.001, t = 3.3, d.f. = 179.4, two-sided), while 15 N 2 O assimilation was consistent between the two biomass types ( p = 0.24, t = −1.2, d.f. = 319.1, two-sided). Fig. 2: Evidence for the direct assimilation of 15 N into biomass from either 15 N 2 or 15 N 2 O. 15 N assimilated into biomass from either 15 N 2 or 15 N 2 O in different months. a Each box shows the 25th to 75th percentiles, horizontal lines the median, open circles denote outliers, and whiskers extend to 1.5 times the interquartile range. b Rates of 15 N 2 assimilation were higher than for 15 N 2 O assimilation in both biomass types. The red dashed line marks the upper threshold for indirect 15 N assimilation if 15 N 2 O was first reduced to 15 N 2 prior to assimilation (see Table 1 ), red shaded area 95% C.I. Data plotted are means ± s.e. Yellow: difference between floating and benthic biomass with 15 N 2 ( p = 0.001, two-sided) , black: difference between 15 N 2 and 15 N 2 O in floating or benthic biomass ( p < 0.001, two-sided). To exclude extreme outliers the data plotted in a and b are 95% of the dataset (2.5–97.5% percentiles). Data in a and b were collected in 5 calendar months for 2 biomass types from 8 to 10 ponds per sampling date ( n = 303 and n = 322 incubations for 15 N 2 and 15 N 2 O treatments, respectively). c No significant production of 15 N 2 from 15 N 2 O in the floating biomass, but d significant production of 15 N 2 in the benthic biomass ( p = 0.04, two-sided). The horizontal line is the mean and shaded area 95% C.I. ( n = 351 incubations for both controls and 15 N 2 O treatments). Full size image To distinguish direct N 2 O fixation (N 2 O → NH 4 + , Eq. 1 ) from indirect fixation i.e., that after an initial reduction of N 2 O to N 2 ([N 2 O → N 2 ] N 2 → NH 4 + , Eq. 2 ) through denitrification, we first checked for any production of 15 N 2 from 15 N 2 O. Overall, the production of 15 N 2 in the 15 N 2 O treatments was not significant in the floating biomass incubations (Fig. 2c ), though 15 N assimilation from 15 N 2 O was significant (Fig. 2b ). In contrast, 30% of the benthic incubations showed measurable 15 N 2 production ( p = 0.04, two-sided, Fig. 2c and Supplementary Fig. 5 ) but with comparable 15 N assimilation from 15 N 2 O (Fig. 2b ). Some denitrification is expected given the sediments recognised capacity to consume oxygen [39] , and our 12 h/12 h light/dark incubation-cycle generated oxygen minima overnight that likely facilitated the reduction of N 2 O to N 2 via denitrification. In addition, we also compared rates of assimilation against a theoretical upper threshold for indirect assimilation of 15 N 2 O after reduction to 15 N 2 (Table 1 and Fig. 2b ). For example, any 15 N 2 from the reduction of 15 N 2 O would be assimilated in proportion to the 15 N-labelling of the total N 2 pool, which would be predominantly ambient 14 N 2 (Table 1 ). As a result, any indirect assimilation of 15 N from 15 N 2 O should have been ~14-fold lower than what we measured in the incubations where we added 15 N 2 directly e.g. 0.8 nmol N g −1 d −1 vs. 11.5 nmol N g −1 d −1 (Table 1 ). In contrast, we measured far higher rates of 5.3 nmol N g −1 d −1 with 15 N 2 O, compared to the upper threshold of 0.8 nmol N g −1 d −1 , on average (0.69 to 0.92 nmol N g −1 d −1 , 95% C.I., Fig. 2b ). Such disproportionately high activity suggests direct assimilation of 15 N from 15 N 2 O into biomass in our freshwater ponds. Table 1 Rationalising N 2 O assimilation as direct N 2 O fixation Full size table Here we added 15 N 2 O to our incubations at concentrations many times higher than atmospheric equilibration (9 µM vs. 0.01 μM) and our rates of 15 N 2 O assimilation are likely upper-potentials. We also characterised the kinetic effect of N 2 O concentration on total N 2 O reduction from 9.2 nM (atmospheric equilibration) to 20,000 nM (Supplementary Fig. 6 ), which enabled us to estimate N 2 O reduction by biomass at in situ concentrations in the ponds. We then scaled these in situ N 2 O reduction estimates by the amount of benthic biomass in the ponds and compared them to our estimates of N 2 O flux into the ponds calculated using our measurements of N 2 O saturation (Fig. 1 and see Supplementary Text 2 ). Accordingly, we estimated in situ N 2 O reduction by the benthic biomass to be −0.75 µmol N 2 O m −2 d −1 (Supplementary Text 2 ) which is equivalent to 56% of the N 2 O flux into the ponds of −1.33 µmol N 2 O m −2 d −1 , on average (range of −3.65 to 0.02 µmol N 2 O m −2 d −1 , including low emissions to the atmosphere in summer). The remaining ~44% of the N 2 O flux is probably driven by microbes associated with the floating biomass (Fig. 2b ) or free-living in the water column [42] and we are confident that our laboratory biomass incubations can rationalise the undersaturation in N 2 O we measured in our ponds. In addition, N 2 flux into the ponds was −3,934 µmol N 2 m −2 d −1 , on average (Supplementary Text 2 ). Multiple fates for total 15 N 2 O reduction Apart from 15 N 2 O being assimilated into biomass and the fraction reduced to 15 N 2 (above), some fixed 15 N 2 O as 15 NH 4 + could potentially “leak” into the pond-water medium to, in turn, be nitrified to 15 NO 2 − and 15 NO 3 − (together 15 NO x − ) – all of which comprise total 15 N 2 O reduction. We characterised total 15 N 2 O reduction and the proportions of the different end-products and found significant 15 N 2 O reduction in the majority (289 out of 372 incubations, 78%) of our incubations enriched with 15 N 2 O. The mean rate of total 15 N 2 O reduction was 364 ± 27 nmol N g −1 d −1 , with the highest rate of total 15 N 2 O reduction occurring in December for both floating (850 ± 178 nmol N g −1 d −1 ) and benthic biomass (784 ± 158 nmol N g −1 d −1 ). To compare summer to winter, we pooled data from November, February and December, for winter, and August and September for summer. Total 15 N 2 O reduction was highest in winter at 507 ± 49 nmol N g −1 d −1 , compared to 237 ± 21 nmol N g −1 d −1 in summer, on average ( p < 0.001, t = −5.1, d.f. = 213.4, two-sided) in both floating ( p < 0.001, t = −5, d.f. = 68.6, two-sided) and benthic ( p = 0.02, t = −2.3, d.f. = 148.5, two-sided) biomass (Fig. 3a ). The patterns in total 15 N 2 O reduction measured in the incubations agreed with the seasonal pattern of N 2 O saturation in the ponds (Fig. 1 ): overall, N 2 O was consumed in both seasons and the ponds were net sinks for N 2 O, with higher N 2 O reduction in winter, corresponding to greater undersaturation in N 2 O in winter. Fig. 3: The fate of total 15 N 2 O reduction in biomass. a Total 15 N 2 O reduction was highest in winter compared to summer in both floating ( p < 0.001, two-sided) and benthic biomass ( p = 0.02, two-sided). Data plotted are means ± s.e. from 95% (2.5% to 97.5% percentiles) of the dataset for summer and winter where n = 180 and n = 160 incubations in summer and winter, respectively (two months for summer, three months for winter). b Production of dissolved inorganic nitrogen in 15 N 2 O incubations. TIN: Total inorganic nitrogen. n = 6 incubations for biomass from 6 ponds. Each box shows the 25th to 75th percentiles, horizontal lines the median, and whiskers extend 1.5 times the interquartile range. c Distribution of the ratio of 15 NO x − production to total 15 N 2 O reduction, dashed line is the median. Data in c are from December, 2020, when the highest rate of total 15 N 2 O reduction was measured ( n = 47 incubation bottles, 5 temperatures with 2 biomass types). d Simplified diagram showing possible pathways for N 2 O reduction in relation to canonical N 2 fixation. Full size image To test whether N 2 O initially fixed intracellularly as NH 4 + (Eq. 1 ) could leak into the water i.e., to be available to the wider ecosystem, we performed additional incubations with samples for nutrient measurements (without formaldehyde, see methods). Although the concentration of NH 4 + was often below the limit of detection for the colorimetric assay (~0.2 μM), the stronger signal for NH 4 + with N 2 O ( p = 0.03) indicated some N 2 O fixed as NH 4 + could “leak”. The concentration of total inorganic nitrogen (TIN) was, on average, 0.32 μM higher in incubations enriched with N 2 O than the controls ( p = 0.001, Fig. 3b ). We also characterised the production of 15 NO x − from 15 N 2 O in December, 2020 (winter), when rates of total 15 N 2 O reduction were highest. The rate of 15 NO x − production was 280 ± 46 nmol g −1 d −1 (mean ± s.e. ), which accounted for 11.7% (median) of total 15 N 2 O reduction (Fig. 3c ). Together, these results show that some N 2 O fixed as NH 4 + can be lost to the water and further oxidised to NO x − through nitrification both of which could be assimilated into PON by the wider community (Fig. 3d ). The temperature dependence of N 2 O fixation As seasonal changes in temperature drove contrasting patterns in N 2 O and N 2 saturation, we characterised the effect of temperature on N 2 O and N 2 reduction by incubating biomass from the ponds at temperatures from 6°C to 25°C. Assimilation of 15 N from 15 N 2 increased at higher temperatures ( p = 0.005, t = 2.8, d.f. = 301, Fig. 4a ), with an estimated Q 10 of 1.38. In contrast, assimilation of 15 N from 15 N 2 O was consistent across all temperatures with no discernible temperature sensitivity. The large variance in Fig. 4a may in part be due to simply normalising the 15 N assimilation data to a unit of dry biomass in each incubation, whereas the communities responsible for N 2 or N 2 O assimilation could be heterogeneous in the biomass samples and across different months of the year. In addition, rates of 15 NO x − production from 15 N 2 O were also consistent across incubation temperatures (Fig. 4b ), which, again, suggested that N 2 O fixation is not sensitive to temperature (i.e., Fig. 4a, b ). Fig. 4: Temperature sensitivity of 15 N assimilation from 15 N 2 and 15 N 2 O and 15 NO x − production from 15 N 2 O. a Temperature sensitivities for 15 N assimilation from 15 N 2 and 15 N 2 O were different ( p = 0.025, two-sided), increasing at higher temperatures for 15 N 2 (slope: 0.35, 95% CI: 0.12–0.5) but 15 N 2 O. As the data were skewed, we used median regression models to minimise bias from outliers. The regression in a , uses the whole dataset but only 95% of the dataset (2.5% to 97.5% percentiles) are presented ( n = 303 and n = 322 for 15 N 2 and 15 N 2 O, respectively, for 5 months, 2 biomass types). b similarly, 15 NO x − production from 15 N 2 O was also invariant to temperature. Data in b are from December, 2020, when total 15 N 2 O reduction was highest ( n = 47 incubations, 5 temperatures, 2 biomass types), blue line is a first-order linear regression, mean ± s.e. 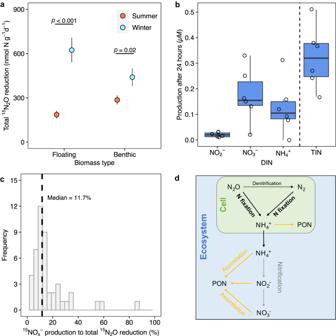Fig. 3: The fate of total15N2O reduction in biomass. aTotal15N2O reduction was highest in winter compared to summer in both floating (p< 0.001, two-sided) and benthic biomass (p= 0.02, two-sided). Data plotted are means ± s.e. from 95% (2.5% to 97.5% percentiles) of the dataset for summer and winter wheren= 180 andn= 160 incubations in summer and winter, respectively (two months for summer, three months for winter).bProduction of dissolved inorganic nitrogen in15N2O incubations. TIN: Total inorganic nitrogen.n= 6 incubations for biomass from 6 ponds. Each box shows the 25th to 75th percentiles, horizontal lines the median, and whiskers extend 1.5 times the interquartile range.cDistribution of the ratio of15NOx−production to total15N2O reduction, dashed line is the median. Data incare from December, 2020, when the highest rate of total15N2O reduction was measured (n= 47 incubation bottles, 5 temperatures with 2 biomass types).dSimplified diagram showing possible pathways for N2O reduction in relation to canonical N2fixation. As the temperature sensitivity of 15 N assimilation and 15 NO x − production was consistent between floating and benthic biomass, the data in a and b have been pooled for both biomass types. Full size image nifH communities in relation to N 2 O reduction The fact that here N 2 O fixation appears less sensitive to temperature than N 2 fixation supported our hypothesis that fixing N 2 O is less energy demanding than fixing N 2 . Here we aimed to address our question of whether N 2 O fixation is mediated by the whole N 2 fixing community or a sub-set, using a long-term incubation with N 2 O-enriched biomass. N 2 O reduction was most rapid during the first 3 days of the incubation and started to decline after the increase in total inorganic nitrogen (TIN, sum of NO 3 − , NO 2 − and NH 4 + ) from 0.44 µM to 0.76 µM and (Fig. 5a and Supplementary Fig. 7a ). We terminated the incubation after 25 days when oxygen production from photosynthesis started to decline (Fig. 5a and Supplementary Fig. 8b ) and characterised the abundance and structure of the nifH community. Fig. 5: Biomass nifH community in relation to N 2 O reduction. a Biomass incubated for 25 days reduced 76 nmol N 2 O-N g −1 (dry weight) on average ( n = 40 incubations for biomass enriched with N 2 O) with activity peaking before inorganic nitrogen accumulated. Data plotted are means ± s.e. b Redundancy analysis (RDA) revealed positive correlations between the initial rates of N 2 O reduction and the relative abundance of 22 nifH OTUs, including 15 Cyanobacterial OTUs and 7 Proteobacterial OTUs (arrows in green). c Heat-map (white to dark red) of the relative abundance of the 22 nifH OTUs (in green), identified in b , in samples (columns, n = 10) in rank order of increasing rate of N 2 O reduction. n = 10 in b and c . N 2 O reduction is presented as a black arrow in b and as a grey ascending triangle in c . Full size image We first tested whether N 2 O reduction was related to the abundance of the whole nifH community (copy numbers of nifH per g wet biomass) but found no relationship ( p = 0.21, F = 1.74, d.f.=18). We then tested whether N 2 O reduction was related to a sub-community by looking for any changes in diversity or composition of the nifH community over the 25-day incubation. Our primers amplified 894 well-represented OTUs ( > 20 reads in at least 3 samples) of which only 227 were identified as nifH OTUs ( see Methods and Supplementary Figs. 9 and 10 ). However, neither the diversity ( p = 0.81, t = 0.24, d.f. = 17.5, two-sided t -statistic tested on the means of Shannon index) nor the composition ( p = 0.99, PERMANOVA, see also Supplementary Fig. 11 for unchanged nifH community composition at 3, 10 and 25 days) of the overall nifH community changed significantly during the 25-day incubation. As an alternative, we used redundancy analysis (RDA) to ordinate the relative abundances of nifH OTUs and the initial rates (i.e., in 10 samples up to day 3) of N 2 O reduction to identify any likely N 2 O fixing candidates (Fig. 5b ). Since N 2 O reduction may be mediated by a subset of the whole nifH community, we relaxed our definition of a well-represented OTU to include <20 reads in at least 3 samples (see Supplementary Fig. 9 ) which retained 72 out of 227 nifH OTUs. Of those 72 OTUs, the relative abundance of 22 were positively correlated with N 2 O reduction i.e., in the ordination their arrows pointed in a similar direction to the arrow for N 2 O reduction. The positive correlations for the 22 OTUs, including 15 Cyanobacteria and 7 Proteobacteria, were further explored by visualising their relative abundance in each biomass sample in rank order of increasing rate of N 2 O reduction (Fig. 5c ). Among the 15 Cyanobacterial OTUs, Pegethrix -like OTU392 and OTU394 (100% identical protein sequence to Pegethrix ) and the Fischerella -like (>99% identical) OTU396 appeared to not only be more common, but they were also more strongly correlated with the initial rates of N 2 O reduction. While OTU412 and OTU389 were also identical to Pegethrix they were either relatively rare or less-well correlated, respectively. Despite the two Methylomonas -like (>99 % identical) Proteobacterial OTU444 and OTU462 being less common than the Cyanobacterial candidates, exisiting in only four samples, their higher relative abundances coincided with higher rates of N 2 O reduction. Moreover, combinations of the five strongest (OTUs 392, 394, 396, 444, 462) N 2 O fixing candidates were not only present in the ten samples used to determine the initial rates of N 2 O reduction but all 40 samples enriched with N 2 O for our 25-day incubation (Supplementary Fig. 9 ). In ecosystems with limited fixed nitrogen (e.g. inorganic NO 2 − , NO 3 − , NH 4 + ), primary production is tightly coupled to N-fixation – typically recognised to be N 2 gas (Eq. 2 ). The undersaturation in N 2 O reported here means that the reduction of N 2 O was greater than its rate of delivery either from the atmosphere or biological sources in the ponds, which shows that these N-limited ponds were overall sinks for N 2 O, including direct N 2 O fixation (Eq. 1 ). Others have argued for direct N 2 O fixation on the premise that if N 2 production was not detected in incubations with N 2 O, then N 2 O fixation was direct [5] , [30] . Here, besides not detecting 15 N 2 production in 76% of our incubations (Fig. 2b ), our disproportionate fixation of N from 15 N 2 O relative to that measured with 15 N 2 provides more substantive evidence for direct N 2 O fixation (Table 1 ). Direct N 2 O fixation represents an alternative to the only widely recognised sink for N 2 O – namely denitrification [6] , [29] . In addition, our estimation of in situ N 2 O fixation helps to rationalise the undersaturation and resultant flux of N 2 O into our ponds (see Supplementary text 2 ). Further, as the scale of N 2 O undersaturation in our ponds (Fig. 1a ) is in line with many other studies also reporting undersaturation in N 2 O in freshwaters (typically ~70–100%) [10] , [16] , [17] , [18] , [21] , this indicates that direct N 2 O fixation could explain the unaccounted for N 2 O undersaturation in many freshwaters [8] , [9] , [10] , [16] , [17] , [18] , [19] , [20] , [21] . We can see similar seasonal trends to what we report here in previous accounts of N 2 O undersaturation. For example, boreal lakes, ponds and rivers show undersaturation in N 2 O which is strongest at coldest temperatures [19] . In Boreal peatlands, N 2 O was undersaturated mostly in spring, increasing to maximum oversaturation in summer, then decreasing to near equilibrium in autumn [46] . From the same study, soils acted as net N 2 O sources at higher temperatures, while most N 2 O sinks occurred below 13 °C [46] . In the surface waters of the Baltic Sea, N 2 O was most undersaturated in winter (December), but was oversaturated in summer and autumn [11] . However, these studies generally lacked a clear explanation for the occurrence and the temperature dependence of N 2 O undersaturation, whereas we now offer an explanation. Our findings demonstrate different temperature dependencies for N 2 and N 2 O fixation. 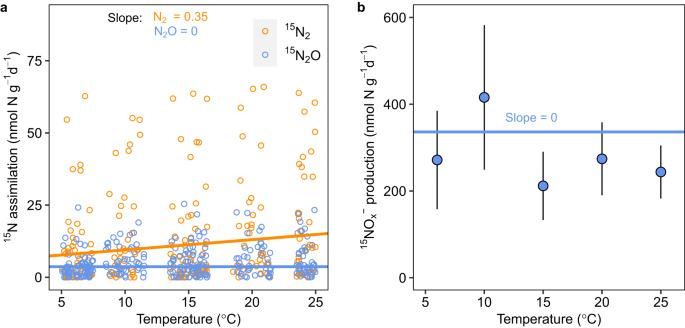Fig. 4: Temperature sensitivity of15N assimilation from15N2and15N2O and15NOx−production from15N2O. aTemperature sensitivities for15N assimilation from15N2and15N2O were different (p= 0.025, two-sided), increasing at higher temperatures for15N2(slope: 0.35, 95% CI: 0.12–0.5) but15N2O. As the data were skewed, we used median regression models to minimise bias from outliers. The regression ina, uses the whole dataset but only 95% of the dataset (2.5% to 97.5% percentiles) are presented (n= 303 andn= 322 for15N2and15N2O, respectively, for 5 months, 2 biomass types).bsimilarly,15NOx−production from15N2O was also invariant to temperature. Data inbare from December, 2020, when total15N2O reduction was highest (n= 47 incubations, 5 temperatures, 2 biomass types), blue line is a first-order linear regression, mean ± s.e. As the temperature sensitivity of15N assimilation and15NOx−production was consistent between floating and benthic biomass, the data inaandbhave been pooled for both biomass types. 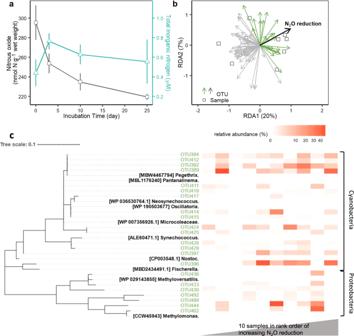Fig. 5: BiomassnifHcommunity in relation to N2O reduction. aBiomass incubated for 25 days reduced 76 nmol N2O-N g−1(dry weight) on average (n= 40 incubations for biomass enriched with N2O) with activity peaking before inorganic nitrogen accumulated. Data plotted are means ± s.e.bRedundancy analysis (RDA) revealed positive correlations between the initial rates of N2O reduction and the relative abundance of 22nifHOTUs, including 15 Cyanobacterial OTUs and 7 Proteobacterial OTUs (arrows in green).cHeat-map (white to dark red) of the relative abundance of the 22nifHOTUs (in green), identified inb, in samples (columns,n= 10) in rank order of increasing rate of N2O reduction.n= 10 inbandc. N2O reduction is presented as a black arrow inband as a grey ascending triangle inc. This difference in N 2 versus N 2 O is supported not only by the opposing seasonal patterns in N 2 and N 2 O saturation in our ponds, but also by the experimentally determined different temperature sensitivities for the assimilation of N 2 and N 2 O by biomass in our incubations. Moreover, the results from our incubations support the seasonal patterns in N 2 and N 2 O saturation in the ponds – with the higher rates of N 2 O reduction in incubations in winter than in summer, matching the stronger N 2 O undersaturation in the ponds in winter, and the elevated temperature effect on N 2 assimilation agrees with that for N 2 saturation in our ponds. Here the apparent lack of temperature sensitivity of N 2 O fixation (Fig. 4 ) suggests that the N-fixing communities may be strongly adapted to substrate limitation (Supplementary Fig. 6 ), with dissolved N 2 O typically at ~10 nM in the ponds compared to ~490 µM for N 2 . This strong kinetic effect of substrate availability on N 2 O fixation has also been reported in incubations with surface seawater [23] and pure culture of marine cyanobacteria Trichodesmium sp [5] . Similar stronger limitation of activity by substrate over temperature is also recognised in other autotrophs such as the methane oxidising methanotrophs [47] , [48] . The contrasting temperature sensitivies of N 2 O and N 2 fixation are probably associated with the energetic advantage of using N 2 O instead of N 2 as a N-substrate for N-fixation [49] . Here we compiled data for studies measuring N 2 fixation in both aquatic and terrestrial ecosystems (Supplementary Fig. 12 and the references cited therein) which clearly shows N 2 fixation increases at higher temperatures. On the other hand, as dissociating the N bond in N 2 O only requires about half of the energy compared to N 2 (refs. [49] , [50] ), N 2 O should be easier to fix at colder temperatures and a higher proportion of total N fixation could be dependent on N 2 O in the cold. For example, with our pond biomass the fraction of total N-fixation coupled to N 2 O at 6°C was 26% higher than that at 25°C (Fig. 4a ). This energy saving offered by fixing N 2 O in the cold might explain why N 2 O undersaturation in our ponds was strongest during the colder months and may also explain the undersaturation reported in cold, boreal environments and Baltic Sea [11] , [19] , [46] . In addition, in northern latitudes cold temperatures typically occur alongside lower light and the ~18% energy saving from fixing N 2 O (Eq. 1 ) compared to N 2 (Eq. 2 ) could provide an over-wintering strategy for a subset of the photosynthetic community. Besides photosynthesis, some chemosynthetic microbes could also benefit. For example, some Methylomonas spp. are known to fix N 2 and were identified here amongst our potential N 2 O fixing candiates. Some 32% of the energy yielded from oxidising CH 4 to CO 2 can be expended on assimilating CH 4 into biomass (equation S6 , Supplementary Text 1 ) with another 56% needed to fix N 2 compared to 47% for N 2 O. Given that methane concentrations are lowest in our ponds in winter [39] - and more widely methane production is known to be tightly coupled to primary production in spring and summer [51] - fixing N 2 O could offer an advantage over N 2 when resources are limited. The concept that N 2 fixation in general is routinely supressed by inorganic N (>~1 µM) has been revised [52] . For example, while there are numerous examples of N 2 -fixing activity being suppressed by inorganic nitrogen in pure cultures of Trichodesmium spp., others have reported its activity in euphotic ocean waters (whole water and Trichodesmium spp. isolates) with ~5 µM to 21 µM NO 3 − (refs. [52] , [53] ), which may indicate short-term tolerance to NO 3 − . In contrast, the N-fixing community in our ponds is exposed to chronic, year round inorganic nitrogen starvation (i.e., <1 µM). Our 25-day incubation showed N 2 O reduction declined after an increase in inorganic nitrogen (NO 3 − and NH 4 + ) to ~0.8 µM (Fig. 5a ), indicating a low-threshold concentration for inorganic nitrogen that apparently limits N 2 O fixation. Such a threshold also reflects the co-occurance of N 2 O undersaturation (Fig. 1a ) with <1 µM inorganic nitrogen throughout the year in our ponds (Fig. 1f ). In contrast, N-rich ecosystems generally act as N 2 O sources [8] , [25] , while N 2 O sinks - mediated through N 2 O fixation – are likely to be found in pristine, cold ecosystems [19] , [21] , [22] , [26] , [27] , [28] . To date, it is not clear which microorganisms are responsible for N 2 O fixation in natural ecosystems. A few studies have reported N 2 O fixation in sea water [5] , [23] and soybean root nodules [30] , but only one study, on pure cultures of the marine cyanobacteria Trichodesmium sp. and Crocosphaera sp., has related the nifH gene to N 2 O fixation [5] . Since being set up in 2005, our nitrogen-limited ponds have developed diverse diazotroph communities [42] , comparable to those in estuaries [54] , freshwater [55] and seawater [56] . Here we set out to link cause to effect by attempting to enrich N 2 O fixing candidates but failed to detect any changes in the total nifH community after 25 days enrichment with N 2 O (Supplementary Fig. 11 ). This might have been due to the decline in rate of N 2 O reduction, as a result of the parallel accumulation in inorganic nitrogen, or longer incubations being needed to detect any change in the total nifH community that is likely slow-growing. In our ordination analysis, five OTUs emerged as the strongest potential candidates for N 2 O fixation i.e., their relative abundance is at least correlated with N 2 O reduction activity. Of these, one is identical to Fischerella , a common diazotroph in freshwater [55] and seawater [57] and also identified in seawater undersaturated in N 2 O [23] and another two being identical to Pegethrix [58] , a newly identified genera of filamentous Cyanobacteria. In addition, proteobacterial methanotrophic diazotrophs have been related to N-fixing activity in N-limited freshwaters [59] , and relatives of our two Methylomonas -like candidates are known to grow on N 2 as their sole nitrogen source [60] . Whether or not our candidate N 2 O-fixers are responsible for the widely reported undersaturation in N 2 O in natural waters needs characterising directly but our first attempt here at least suggests N 2 O fixation is likely mediated by a subset of diazotrophic communities. In addition, our work shows that N 2 O fixation can occur in an abundance of N 2 i.e., against the high natural N 2 background. This indicates that N 2 O fixation could happen in natural ecosystems replete in N 2 and provides further insight into the communities responsible for N 2 O fixation. For example, nifH communities could fix N 2 and N 2 O randomly, with the ratio of N 2 O to N 2 fixation being simply proportional to the relative availability of N 2 O to N 2 . However, the distinct seasonal patterns we measured for N 2 and N 2 O undersaturation (Fig. 1 ), coupled to disproportionate rates of N 2 O fixation (Fig. 2 ) and higher proportion of N 2 O fixation at colder temperatures (Fig. 4a ) - all indicate that a specialised subset of the nifH community (Fig. 5 ) likely favoured N 2 O over N 2 at colder temperatures in support of our nifH ordination analysis. To put our estimates of N fixation into an ecological context, we compared estimates of the N 2 flux (Supplementary Text 2 ) with former estimates of gross primary production (GPP) in the ponds [40] . For example, the average net N 2 flux into the ponds was 3934 µmol N 2 m −2 d −1 , which, assuming Redfield ratios of 106:16 for C:N, could sustain GPP of 52,126 µmol C m −2 d −1 and which is comparable to GPP measured previously of 51,488 to 70,792 µmol C m −2 d −1 (ref. [40] ). Moreover, the seasonal dynamics in N 2 flux in our study also matched that of GPP reported previously [40] , with both peaking in the summer (Fig. 1b ). In contrast, while the flux of N 2 O is comparatively minor (~0.03 %) in terms of supporting GPP, it is great enough to maintain a strong sink for N 2 O. To date, denitrification in either anoxic or oxic-to-anoxic transitioning waters is still the only widely recognised sink for N 2 O [6] , [7] , [29] . Here, as an alternative to denitrification, direct N 2 O fixation can rationalise the undersaturation in N 2 O in our ponds and could also explain the various unaccounted for N 2 O sinks – of similar magnitude – reported in natural, pristine waters [10] , [17] , [19] , [21] , [22] , [28] , [46] . As N 2 O undersaturation is favoured in the cold, rising temperatures could erode this natural sink for such a potent climate-gas. Nutrient analysis Temperature and O 2 were measured in each pond using HQD portable metre (Hach). Samples of water for nutrient analysis were filtered (0.45 μm PES, 25 mm, pre-washed with deionized water) into Falcon tubes, kept cool and frozen at −20 °C back in the laboratory. Samples were thawed overnight at 4 °C and analysed by standard wet-chemistries for NO 2 − , NO 3 − , NH 4 + and SRP on an autoanalyzer (San ++ , SKALAR Analytical B.V.) [61] against certified reference materials, traceable to NIST. The limits of detection were 0.05 μM and 0.1 μM for NO 2 − and NO x − (NO 2 − + NO 3 − ), respectively, 0.2 μM for NH 4 + and 0.05 μM for SRP. SRP and total inorganic nitrogen (TIN, NO 3 − + NO 2 − + NH 4 + ) below detection limits were omitted from any calculations. Dissolved N 2 and N 2 O in the ponds For dissolved N 2 and N 2 O analyses, water samples were taken carefully at mid-water-depth (~20 cm from the surface) from each pond using a 60 mL syringe and tubing. Five gas-tight vials (12 mL Exetainer, Labco, two vials for N 2 O and three for N 2 ) for each pond were allowed to overflow three times, preserved with ZnCl 2 (50 μL of 50% w/v) [62] , closed and mixed by hand. Extra pond water samples for reference N 2 saturation were collected and preserved along with samples of air. In a temperature-controlled laboratory at 22 °C, references for N 2 saturation were prepared by equilibrating the pond water with the laboratory air, and then water and air samples were collected as for the field samples. Helium headspaces (2 mL 99.999% purity) were created in all sample and reference vials, followed by 24 h equilibration on an orbital shaker (SSL1, Stuart) in the same laboratory and all vials weighed to determine the exact volume of headspace and water. For N 2 O, 100 μL of sample headspace was injected by an autosampler into a gas chromatograph fitted with a µECD (Agilent Technology UK Ltd., South Queensferry, UK) along with air samples using conditions described previously [63] . Calibration was performed against known concentrations of N 2 O from a NOAA standard (traceable to the SI unit “amount of substance fraction”) at 359.73 ppb or 120 ppb and 1.04 ppm and 96 ppm from BOC, UK, cross-calibrated to the NOAA standard. The precision for N 2 O concentration was 2% (coefficient of variation, n = 10). The total concentration of N 2 O in each vial was calculated using solubility coefficents [64] as described before [63] and the degree of over- or under-saturation calculated by comparison to the expected concentration of N 2 O for pond water at equilibrium with the atmosphere (see Supplementary Fig. 1 ). For N 2 analysis, we used the published N 2 :Ar method [65] . 100 μL of headspace was injected by an autosampler into an elemental analyzer, (Flash EA 1112 series, Thermo Finnigan) to remove O 2 by the hot-copper reduction, before passing to a continuous flow isotope ratio mass spectrometer (CF-IRMS, Delta V Plus, Thermo Finnigan). Throughout each run, air samples were analysed to correct for drift and the expected concentrations for N 2 or Ar in the headspace (C hs ) calculated using the solubility of N 2 and Ar for air at both field (K field ) and laboratory (K lab ) temperature [66] : 
    _×_+_×K_lab×_=_×_×_
 (4) Where V hs and V aq are the volumes of headspace and water in a vial and C hs and C field the concentration of either gas in the headspace or field air, respectively. The saturation of N 2 in the samples was then derived by comparing the measured to expected ratio of N 2 to Ar in the samples to that in the pond water ref. [67] : 
    _2(%)=(_2/ /_2/ )_/(_2/ /_2/ )_× 100
 (5) Precision for the ratio of N 2 to Ar for triplicate reference water and air standards was 0.1% and 0.05% (coefficient of variation), respectively. We also tested the effect of calculating N 2 saturation with different references, with the ratio for deionized versus pond water being 99.7% and 99.82%, on average ( n = 20 and n = 8, respectively). Biomass incubations to characterise N 2 and N 2 O fixation Two types of biomass were collected from the ponds for the routine (24-h) incubations (Supplementary Fig. 3 ) and see below for the 25-day incubation. Floating assemblages on the ponds, comprising Oedogonium spp. and microorganisms attached to the filaments (Supplementary Fig. 3b ) and green or yellow benthos assemblages (Supplementary Fig. 3c ), sampled avoiding the sandy sediments beneath. Samples of biomass were collected in sterile Falcon tubes (50 mL) and transported back to the laboratory in a cool box and stored overnight at 15 °C before preparing the incubations. Despite the ponds being low in dissolved inorganic nitrogen, we standardised nutrient concentrations in the incubations by using an artificial pond water medium devoid of fixed N comprising: CaCl 2 (0.5 mM), KCl (1 mM), MgSO 4 (0.25 mM), KHCO 3 (0.7 mM) and NaHCO 3 (0.5 mM) in deionized water. P was added to 0.08 μM of NaPO 4 , based on measured SRP concentrations in the ponds. Incubations of biomass with 15 N 2 and 15 N 2 O tracers Floating or benthic biomass was weighed (~3 g wet weight) into 12 mL gas-tight vials and, for the 15 N 2 O treatment, filled with oxygen-saturated artificial pond water and closed. 100 μL of water was replaced by 15 N 2 O stock solution (see below) with a gastight syringe. For the 15 N 2 treatment, each vial was filled with 10 mL of oxygen-saturated artificial pond water and 2 ml of 15 N 2 stock and closed (see below). All incubations were prepared without a headspace to ensure 15 N-substrate concentrations were the same under different temperatures. Parallel controls were prepared in the same way without either 15 N-gas. T 0 (Time zero) vials were killed with 200 μL of 50% (w/v) formaldehyde immediately and the remainder incubated in temperature-controlled orbital incubators (SI500, Stuart at 50 cycles min −1 ) at 6, 10, 15, 10 and 25 °C on a 12 h light/12 h dark cycle for 24 h. Time final (T f ) samples were killed as above, brought to 22 °C, helium headspaces created in all vials, and all allowed to equilibrate for 24 h, as above. Stock solutions for 15 N 2 and 15 N 2 O additions to the biomass incubations To avoid the recognised equilibration problems with the 15 N 2 “bubble method”, especially during short-term incubations [68] , we first made an aqueous 15 N 2 stock with the artificial pond water. 200 mL of artificial media were injected into a 0.5 L gas sampling bag along with 40 mL 15 N 2 gas (98% atom % 15 N, Sigma-Aldrich) and allowed to equilibrate for 24 h while gently rocking. 15 N 2 O stock solutions were prepared by replacing 3 mL of water with 15 N 2 O gas (98% atom % 15 N, Cambridge Isotope Laboratories, Inc.) in a 50 mL sealed serum bottle. The solubility of N 2 is low and to maximise 15 N 2 labelling we added a relatively large amount (~2 ml) of 15 N 2 stock solution to the 12 mL vials (~16% v/v). To keep the dissolved nutrients and gases at background levels in the 15 N 2 treatments -and the same as in the controls and 15 N 2 O treatment- we used artificial freshwater medium instead of deionized water for preparing 15 N 2 stocks. In contrast to N 2 , N 2 O is highly soluble, with only ~100 μL of 15 N 2 O stock being needed in each treatment (~0.8% v/v) to reach the comparable concentration of 15 N-N 2 addition (~10 μM). 15 N 2 O and 15 N 2 stocks were prepared fresh before each experiment and their respective dosages tested by spiking controls. Characterising total 15 N 2 O reduction The concentration of 15 N 2 O in the samples was measured on a CF-IRMS (Delta V Plus, Thermo-Finnigan) with an automated trace gas pre-concentrator (PreCon, Thermo-Finnigan) [63] . A sub-sample from the headspace of each sample was transferred to a 12 mL air-filled gas-tight vial. The high 15 N-labelling of 15 N 2 O (on average, 97.7% of 46 N 2 O) in the 15 N 2 O treatment meant only a small aliquot of sample (10 μL) was needed to keep the signal within the measurable range of 46 N 2 O. Mass-to-charge ratios were measured for m/z 44, 45 and 46 and the concentration of N 2 O determined by calibration against known amounts (0.02–2 nmol) of natural abundance N 2 O (96 ppm N 2 O standard, BOC, UK) [63] . Note, whether the mass spectrometer is calibrated with high purity 15 N 2 O or natural abundance N 2 O, the signal-to-mole ratio is constant (Supplementary Fig. 13 ). Here the concentration of total 15 N 2 O is expressed as 15 N 2 O = 45 N 2 O + 2 × 46 N 2 O and the reduction of 15 N 2 O calculated by subtracting 15 N 2 O concentrations in T f samples from T 0 samples. Characterising any dissimilatory reduction of 15 N 2 O to 15 N 2 Any production of 15 N 2 in the 15 N 2 O treatments was measured by the CF-IRMS (Delta V Plus, Thermo Finnigan), after bypassing the copper reduction step to avoid reduction of 15 N 2 O to 15 N 2 (ref. [69] ). The concentration of total N 2 was calculated from the solubility of N 2 (ref. [66] ) and the signal of total N 2 mole masses i.e., m/z 28, 29 and 30 in the samples and air standards [70] . Drift in m/z 30 was corrected by inserting air standards for every 10 samples. Changes in the concentration of 15 N 2 (Δ 15 N 2 , nmol N d −1 ) were calculated by the excess 15 N 2 in 15 N 2 O treatments compared to the controls, where Δ 15 N 2 = Δ 29 N 2 + 2 x Δ 30 N 2. The limit of detection for Δ 15 N 2 in the incubations is ~0.14 μM. Characterising assimilation of 15 N 2 O or 15 N 2 into biomass After all the gas measurements, samples were centrifuged and the supernatants filtered (as above). The remaining biomass was dried, homogenised and sub-samples weighed into tin caps (6 × 4 mm, Elemental Microanalysis) for elemental analysis as described previously [41] . The level of 15 N enrichment in biomass incubated with either 15 N 2 or 15 N 2 O was then calculated by the difference in excess 15 N atom % relative to the controls, where excess 15 N atom % is the difference in 15 N atom % between T 0 and T f in the 24-h incubations: 
    ^15N enrichment=(excess^15N atom%)_Treatment-(excess^15N atom%)_Control
 (6) Rates of 15 N assimilation (nmol 15 N g −1 day −1 ) by biomass into particulate organic nitrogen (PON) were calculated as: 
    ^15N assimilation rate=PON×^15N enrichment/(t×dw)
 (7) Where PON is particulate organic nitrogen in a sample of biomass, \(\Delta {{\mbox{t}}}\) is the incubation time (24 h), and dw the dry weight (g). Characterising 15 N 2 O fixation As total 15 N 2 O reduction includes both assimilatory 15 N 2 O fixation and dissimilatory 15 N 2 O reduction to 15 N 2 , total 15 N 2 O fixation can be calculated by subtracting 15 N 2 production from total 15 N 2 O reduction: 
    Total^15N_2O fixation=Total^15N_2O reduction-^15N_2 production
 (8) Where total 15 N 2 O fixation includes 15 N 2 O assimilated into biomass, as well as any fixed 15 N 2 O present in the pond water medium as dissolved inorganic nitrogen ( 15 DIN, e.g., 15 NH 4 + , 15 NO 2 − and 15 NO 3 − ): 
    Total^15N_2O fixation=^15N_2O assimilation+^15DIN production
 (9) We characterised any 15 DIN production coupled 15 N 2 O fixation by measuring 15 NO x − (i.e., 15 NO 3 − + 15 NO 2 − ) with sulfamic acid [62] , testing for any effect of formaldehyde on the 15 NO x − assay (Supplementary Fig. 14 ). Due to the high 15 N 2 O background, it was not possible to measure any 15 NH 4 + from 15 N 2 O using the sensitive sodium-azide assay as it converts 15 NO 2 − to 15 N 2 O. Further, as the formaldehyde preservative interferes with the colorimetric NH 4 + assay, we did additional incubations in October 2021 without formaldehyde, following the exact incubation procedure described above. Here, samples for DIN were immediately centrifuged and frozen at −20 °C while parallel samples for gases were treated as above. Concentrations of DIN in controls and 15 N 2 O treatments were measured by the automated wet-chemistry autoanalyzer ( see ‘Nutrient analysis’ in Methods), while changes in N 2 O concentrations were measured by GC/µECD [63] . nifH communities in relation to N 2 O reduction over a 25-day incubation To characterise any nifH communities potentially involved in N 2 O fixation, we incubated floating biomass from the ponds with excess N 2 O for as long as possible, looking either for changes in the nifH community or relationships between particular nifH families and N 2 O reduction. Floating biomass was collected from 10 ponds in May 2021 (as above) and once back in the laboratory kept in a temperature-controlled room at 15°C overnight. The next day, 7 g wet biomass was transferred into 70 mL serum bottles ( n = 80, 8 serum bottles per pond), filled with water and sealed. N 2 O stock solution (600 µL as above) was injected into half of the serum bottles, while venting water through a needle, to create an initial N 2 O concentration of ~10 µM and the remaining serum bottles left unamended as controls. Temperature-controlled incubations were carried out on a 12 h:12 h light/dark cycle as above. A total of 20 serum bottles (10 with N 2 O and 10 controls) were sacrificed after 0, 3 and 10 days of incubation, respectively, while the last 20 serum bottles were incubated until the daily maximum in oxygen started to decline. Oxygen was measured with optical sensors (OXSP5, FireSting®, Pyro Science GmbH, Germany) at ~2-hourly intervals after lights and the incubations terminated on day 25 when daily maximum oxygen started to decline (Supplementary Fig. 8 ). Sub-samples of water were transferred from each serum bottle into a 3 ml gas-tight vial (Exetainers, Labco) after 0, 3, 10 and 25 days of incubation, fixed with 50 µl formaldehyde, sealed and stored at room temperature. After creating a helium headspace N 2 O concentrations were measured by GC/µECD (as above). The remaining water was filtered and frozen at −20 °C for later quantification of NO 3 − , NO 2 − and NH 4 + , as above. Biomass was frozen at −20 °C until DNA extraction (June 2021) from ~0.5 g of wet biomass (DNeasy PowerSoil kit, Qiagen) as per the manufacturer’s instructions. nifH gene abundance (qPCR) and library preparation Gene abundance of nifH was determined using qPCR with IGK3/DVV (forward, 5’-GCIWTHTAYGGIAARGGIGGIATHGGIAA-3’; reverse, 5’- ATIGCRAAICCICCRCAIACIACRTC-3’) [71] using a CFX384 Touch Real-Time PCR (Bio-Rad) in 10 µL reactions containing 5 µL SensiFAST SYBR No-ROX mastermix (Meridian Bioscience), 0.8 µL of each primer (10 µM), 0.8 µL DNA template and 2.6 µL molecular biology quality water (MBQW). The qPCR programme was 98 °C (3 min) then 40 cycles of 98 °C (15 s), 58 °C (60 s), 72 °C (60 s). Standard curves (10 5 to 10 8 copies per µL) were prepared from plasmid DNA containing nifH and product specificity confirmed by endpoint melt curve analysis. A three step PCR was used to prepare the nifH library [72] . nifH was amplified using IGK3/DVV in 10 µL of MyTaq Red Mix (Bioline), 0.8 µL of each primer (10 µM), 0.8 µL of DNA template and 7.6 µL MBGW on a T100 Cycler (Bio-Rad) at (1) 94 °C (5 min); (2) 36 cycles of 94 °C (30 s), 57 °C (45 s), 72 °C (30 s); (3) 72 °C (10 min). These PCR products were then re-amplified with IGK3/DVV appended with overhang MiSeq adaptors in 25 µL containing 12.5 µL of MyTaq Red Mix (Bioline), 1 µL of each primer (10 µM), 1 µL of amplicons from the first step as template and 9.5 µL of MBGW. The PCR programme was: (1) 94 °C (4 min); (2) 12 cycles of 94 °C (30 s), 57 °C (45 s), 72 °C (30 s); (3) 72 °C (7 min). PCR products were cleaned using AMPure XP beads and multiplexing barcodes added by the Index PCR in 25 µL containing 12.5 µL of MyTaq Red Mix (Bioline), 0.5 µL of each primer (10 µM), 0.5 µL of DNA template and 11 µL of MBQW at (1) 95 °C (3 min); (2) 8 cycles of 98 °C (20 s), 57 °C (15 s), 72 °C (15 s); (3) 72 °C (5 min). Final amplicons were quantified (Qubit 2.0 Fluorometer (Invitrogen)) and normalised to 4 nM (SequalPrep Normalization Plate Kit, Invitrogen), combined and sequenced (Illumina MiSeq, 300 base paired-ends). Sequence processing pipeline and phylogenetic analysis Paired-end de-multiplexed files were imported into QIIME2 (v.2021.11) on the Apocrita HPC facility at Queen Mary University of London [73] (Supplementary Fig. 9 ) and processed using DADA2 to trim primers, remove low-quality sequences and chimeras [74] . Sequences were clustered into species-level OTUs at 95% similarity [72] , singletons and sequences >356 bp or <333 bp and low-abundance OTUs (<20 reads and in 3 samples or less) were removed. Amino acid sequences were aligned to known nifH and non- nifH references and a phylogenetic tree constructed using COBALT [75] . The primers IGK3/DVV can amplify non- nifH homologues including the chlorophyll synthesis genes BChL and ChlL and these were identified after translating the OTU sequences using “Translate” in MEGA (version 10.2.2). Translation initiation site adjustment and frameshifts were detected using blastp [76] . Amino acid sequences were aligned to known nifH and non- nifH references and a phylogenetic tree constructed using COBALT [75] . The non- nifH OTUs were identified using distinct non-conservative short sequence motifs and visualised using the iTOL tool [77] that appeared as two separate clusters on the phylogenetic tree ( see Supplementary Fig. 10 ). Approximately 82% of the sequences were non- nifH homologues, which is common when using general nifH - primers [71] . Non- nifH sequences were removed and q-PCR estimates of nifH gene abundances were corrected for the proportion of non- nifH sequences in each sample. Statistical analysis Statistical analysis and plotting were performed in R [78] using RStudio (Version 1.3.1093). We used generalised additive mixed effects models (GAMMs) [79] to characterise the seasonal patterns in N 2 and N 2 O saturation, fitting sampling month as a fixed effect and each replicate pond as random effects. We included an interaction term for sampling month by gas (N 2 or N 2 O) to explore any distinct seasonality in N 2 and N 2 O saturation. Models were ranked by the small sample-size corrected Akaike Information Criterion (AICc) using the ‘MuMIn’ package (Supplementary Table 1 ). Rate data for total 15 N 2 O reduction and 15 N assimilation were skewed, potentially due to normalising to unit dry biomass which may not account for the true abundance of N 2 and N 2 O fixers. Therefore, we present 95% of data (2.5% to 97.5% percentiles) for both datasets (Figs. 2 a, c, 3 a and 4a ) and fitted quantile regression models (‘quantreg’ [80] ) rather than mean regression models to the full dataset for rate of 15 N assimilation to minimise any bias from outliers (median regression lines, Fig. 4a ). The difference between the temperature response of 15 N 2 and 15 N 2 O was compared using the ‘emmeans’ package. nifH Shannon diversity was calculated using the ‘estimate_richness’ function in the ‘phyloseq’ package [81] and any changes in the nifH community calculated using the ‘adonis’ function from the ‘Vegan’ package [82] (with Original UniFrac distance). Principal Coordinates Analysis (PCoA) was used to test the significance of either incubation day or excess N 2 O on nifH community composition by Permutational multivariate analysis of variance (PERMANOVA) and redundancy analysis (RDA) to ordinate N 2 O reduction and nifH relative abundance. Reporting summary Further information on research design is available in the Nature Portfolio Reporting Summary linked to this article.